Rnd3 coordinates early steps of cortical neurogenesis through actin-dependent and -independent mechanisms The generation of neurons by neural stem cells is a highly choreographed process that requires extensive and dynamic remodelling of the cytoskeleton at each step of the process. The atypical RhoGTPase Rnd3 is expressed by progenitors in the embryonic brain but its role in early steps of neurogenesis has not been addressed. Here we show that silencing Rnd3 in the embryonic cerebral cortex interferes with the interkinetic nuclear migration of radial glial stem cells, disrupts their apical attachment and modifies the orientation of their cleavage plane. These defects are rescued by co-expression of a constitutively active form of cofilin, demonstrating that Rnd3-mediated disassembly of actin filaments coordinates the cellular behaviour of radial glial. Rnd3 also limits the divisions of basal progenitors via a distinct mechanism involving the suppression of cyclin D1 translation. Interestingly, although Rnd3 expression is controlled transcriptionally by Ascl1, this proneural factor is itself required in radial glial progenitors only for proper orientation of cell divisions. The generation of neurons by stem cells involves cellular movements, cell divisions and dynamic changes in cell–cell interactions. How these different steps of neurogenesis, which all require extensive cytoskeleton rearrangement, are coordinately regulated and coupled to the activation of a neurogenic programme of gene expression is not well understood. The neural stem cells of the embryonic brain or radial glial cells are highly polarized cells that are attached to one another in the ventricular zone (VZ) of the brain by apically located adherens junctions. Their nuclei migrate during the cell cycle from a basal position during S phase to an apical position during mitosis, and the nuclei of the daughter cells migrate back to enter S phase on the basal side of the VZ, in a process of interkinetic nuclear migration (INM). During the peak of neurogenesis, most radial glial cells divide asymmetrically with vertical cleavage planes. In these divisions, one daughter remains a radial glial cell and continues to divide at the ventricular surface, whereas the other loses its apical attachment and exits the cell cycle either immediately or after one or a few divisions as a basal progenitor [1] , [2] , [3] . Fewer radial glial cells undergo oblique or horizontal divisions, and these divisions have been proposed to generate outer radial glial [2] , [4] . The actin cytoskeleton has an important role in both the positioning of the mitotic spindles [5] and the formation and remodelling of adherens junctions [6] , [7] . Actin has also been implicated in the regulation of INM [8] , [9] , [10] , [11] as well as other cortical progenitor behaviours [12] , [13] , [14] . Members of the small RhoGTPase superfamily, which have important roles in the regulation of the actin cytoskeleton, are involved in the coordination of the different steps of neurogenesis. Cdc42 activity is essential for the maintenance of apical adheren junction and for INM [15] , [16] . RhoA signalling has also a role in the maintenance of adherens junctions and in apico-basal polarity [17] , [18] , [19] , in the orientation of mitotic cleavage planes [20] , [21] and in progenitor proliferation [22] . Rac1 is required in neural progenitors for proper interkinetic nuclear movement, cytokinesis and cell-cycle re-entry [23] , [24] , [25] . We have previously shown that the small GTP-binding protein Rnd3 regulates the migration of cortical neuron downstream of the proneural protein Ascl1 by promoting the disassembly of actin filaments [26] . Because Rnd3 is also expressed in cortical progenitors [26] , we have asked whether it is also involved in earlier steps of neurogenesis that also require regulation of the actin cytoskeleton. We show here that Rnd3 regulates the movements of the nuclei of radial glial cells during INM, that it exerts a control over the orientation of mitotic spindles and that it is required for the maintenance of adherens junctions. As for its function in migrating neurons [26] , Rnd3 regulates these early steps of neurogenesis by inhibiting actin filament polymerization. Rnd3 also limits the divisions of basal progenitors, but, interestingly, this involves a distinct mechanism of suppression of cyclin D1 translation. Our results thus reveal that Rnd3 exerts its pleiotropic functions in early steps of cortical neurogenesis by employing distinct mechanisms in radial glial cells and basal progenitors. Rnd3 is required for INM To assess the function of Rnd3 in cortical progenitors, we silenced the gene in the cortex of E14.5 embryos by in utero electroporation of a construct co-expressing Rnd3 short hairpin RNA (shRNA), or scrambled shRNA in control experiments, and GFP to identify electroporated cells. Twenty-four hours later, we traced a cohort of cortical progenitors by labelling them in S phase with 5-bromo-2′-deoxyuridine (BrdU) and examining their positions after 30 min, 3 h or 6 h ( Fig. 1a ). Thirty minutes after the pulse, nuclei that had incorporated BrdU had undergone INM and had migrated from the basal to the apical side of the VZ ( Fig. 1b ). Quantification of the distribution of VZ progenitors co-labelled for GFP and BrdU revealed that the nuclei of progenitors electroporated with the Rnd3 shRNA had migrated less than the nuclei of progenitors electroporated with the control shRNA, and a larger fraction of them remained on the basal side of the VZ ( Fig. 1c ). Three hours after the pulse, some control BrdU + , GFP + cells had divided, and one of the daughters had already moved out of the VZ, whereas the nucleus of the radial glial daughter had moved back towards the basal side of the VZ ( Fig. 1d ). In contrast, Rnd3- silenced cells that were delayed in their basal–apical movement had just divided at the ventricular surface, leading to an accumulation of cells at the ventricular surface ( Fig. 1e ). Altogether, these results indicate that silencing Rnd3 in cortical progenitors impairs INM. 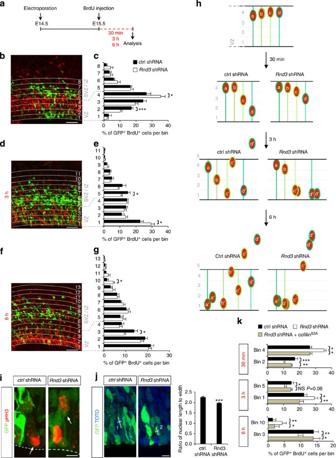Figure 1: Rnd3 regulates INM of cortical neuron progenitors by depolymerizing F-actin. (a) Protocol used to study INM. Cerebral cortices from E14.5 embryos were electroporatedin uterowithRnd3shRNA or control (ctrl) shRNA, and subjected 24 h later to 30 min, 3 h or 6 h BrdU pulse labelling, followed by fixation and co-immunostaining for GFP (green) and BrdU (red). (b,d,f) Distribution of GFP+BrdU+cells after 30 min (b), 3 h (d) or 6 h (f) BrdU pulse across the VZ, SVZ and IZ, divided into bins as indicated, with bin 1 being at the ventricle surface and bin 4 at the VZ–SVZ boundary. (c,e,g) GFP+BrdU+cells in a given bin are expressed as percentage of the total number of GFP+BrdU+-labelled cells in all bins. Data are presented as the mean±s.e.m. from seven sections prepared from four embryos obtained from two or three litters. Student’st-test; *P<0.05 and ***P<0.001. (h) Schematic representation of the results obtained inb–g. (i) Illustration of a mitotic radial glial cell dividing along or away from the ventricular surface (dashed line) 24 h after ctrl orRnd3shRNA electroporation, respectively, at E14.5. GFP identifies electroporated cells and phosphohistone H3 (pHH3) in red marks mitotic cells. (j) Quantification of the ratio of nuclear length-to-width (indicated by white lines on the pictures; cell 1 ratio>cell 2 ratio) in GFP+cells 24 h after electroporation (E14.5) of ctrl orRnd3shRNA.n=163 cells for ctrl shRNA,n=162 cells forRnd3shRNA from 10 sections prepared from four embryos obtained from two or three litters; mean±s.e.m; Student’st-test; ***P<0.001. (k) Co-electroporation of cofilinS3A, a non-phosphorylatable form of cofilin that depolymerizes F-actin, fully rescues the defects observed afterRnd3silencing. Quantification is similar toc,eandg. Mean±s.e.m; one-way analysis of variance followed by a Fisher’s protected least significant differencepost-hoctest; *P<0.05, **P<0.01 and ***P<0.001. Scale bar, 50 μm (b,d,f) and 5 μm (i,j). See also Supplementary Figs S1, S2, and S4. NS, not significant. Figure 1: Rnd3 regulates INM of cortical neuron progenitors by depolymerizing F-actin. ( a ) Protocol used to study INM. Cerebral cortices from E14.5 embryos were electroporated in utero with Rnd3 shRNA or control (ctrl) shRNA, and subjected 24 h later to 30 min, 3 h or 6 h BrdU pulse labelling, followed by fixation and co-immunostaining for GFP (green) and BrdU (red). ( b , d , f ) Distribution of GFP + BrdU + cells after 30 min ( b ), 3 h ( d ) or 6 h ( f ) BrdU pulse across the VZ, SVZ and IZ, divided into bins as indicated, with bin 1 being at the ventricle surface and bin 4 at the VZ–SVZ boundary. ( c , e , g ) GFP + BrdU + cells in a given bin are expressed as percentage of the total number of GFP + BrdU + -labelled cells in all bins. Data are presented as the mean±s.e.m. from seven sections prepared from four embryos obtained from two or three litters. Student’s t -test; * P <0.05 and *** P <0.001. ( h ) Schematic representation of the results obtained in b – g . ( i ) Illustration of a mitotic radial glial cell dividing along or away from the ventricular surface (dashed line) 24 h after ctrl or Rnd3 shRNA electroporation, respectively, at E14.5. GFP identifies electroporated cells and phosphohistone H3 (pHH3) in red marks mitotic cells. ( j ) Quantification of the ratio of nuclear length-to-width (indicated by white lines on the pictures; cell 1 ratio>cell 2 ratio) in GFP + cells 24 h after electroporation (E14.5) of ctrl or Rnd3 shRNA. n =163 cells for ctrl shRNA, n =162 cells for Rnd3 shRNA from 10 sections prepared from four embryos obtained from two or three litters; mean±s.e.m; Student’s t -test; *** P <0.001. ( k ) Co-electroporation of cofilin S3A , a non-phosphorylatable form of cofilin that depolymerizes F-actin, fully rescues the defects observed after Rnd3 silencing. Quantification is similar to c , e and g . Mean±s.e.m; one-way analysis of variance followed by a Fisher’s protected least significant difference post-hoc test; * P <0.05, ** P <0.01 and *** P <0.001. Scale bar, 50 μm ( b , d , f ) and 5 μm ( i , j ). See also Supplementary Figs S1, S2, and S4. NS, not significant. Full size image Defects in the cell-cycle progression of progenitors have been shown to interfere with INM [27] , [28] . However, the duration of the different phases of the cycle was unaffected by Rnd3 silencing ( Supplementary Fig. S1a–d ), indicating that Rnd3 directly regulates the INM of cortical progenitors. Conversely, blocking of INM during apical nuclear migration in G2 does not prevent cell-cycle progression and results in ectopic mitoses [27] , [29] . Accordingly, we observed progenitor cells dividing a short distance away from the ventricular surface 1 day after Rnd3 shRNA electroporation but not after control shRNA electroporation ( Fig. 1i ). Nuclei undergoing INM normally have an elongated morphology, and INM impairment results in nuclei adopting a more rounded shape [30] , [31] , [32] . We measured the length-to-width ratio of nuclei of transfected progenitors and observed that Rnd3 -silenced progenitors have significantly less-elongated nuclei ( Fig. 1j ). Together, these results indicate that Rnd3 is required for normal INM of cortical neuron progenitors. To determine whether Rnd3 acts by regulating actin depolymerization in VZ progenitors as in migrating neurons [26] , we co-electroporated Rnd3 shRNA with cofilin S3A , a non-phosphorylatable form of cofilin that constitutively depolymerizes F-actin. Cofilin S3A fully rescued the INM defects of Rnd3 -silenced progenitors ( Fig. 1k and Supplementary Fig. S2 ), thus demonstrating that Rnd3 regulates INM of cortical progenitors by promoting F-actin depolymerization. BrdU-pulsed cortices were also examined 6 h later, at which time some BrdU + cells had left the VZ and migrated in the subventricular zone (SVZ) and intermediate zone (IZ) in control experiments ( Fig. 1f and Supplementary Fig. S1e ). Rnd3 silencing increased the fraction of BrdU + cells that reached the SVZ and IZ and reduced the fraction that remained in the VZ ( Fig. 1g and Supplementary Fig. S1e ), suggesting that Rnd3 activity regulates not only INM in the VZ but also the movement of cells out of the VZ. This distinct function is examined in the next section. Rnd3 controls cleavage-plane orientation Radial glial cells in the cortical VZ divide mostly with a vertical cleavage plane, and their two daughter cells remain attached to the ventricular surface immediately after mitosis [1] , [2] . When a progenitor divides with an oblique or horizontal cleavage plane, one of its daughters lacks an apical process attached to the ventricular surface and migrates away from the VZ. The increase in number of cells located outside of the VZ after Rnd3 knockdown ( Fig. 1g ) therefore suggested that cleavage planes might be abnormally oriented, resulting in cells detaching prematurely from the ventricular surface. In control experiments, cleavage planes at metaphase and anaphase–telophase were mainly vertical, and horizontal or oblique cleavage planes were relatively rare (8.6% and 17.9%, respectively; Fig. 2c ) as previously observed [1] , [33] , [34] . When Rnd3 was knocked down, the fraction of cells dividing with an oblique or horizontal cleavage plane increased significantly (to 57.7% and 37.5%, respectively; Fig. 2c ). The increase in divisions with non-vertical cleavage planes might account for the increased fraction of Rnd3 -silenced, BrdU-labelled cells that migrate out of the VZ 6 h after the BrdU pulse ( Fig. 1g ). Like INM, orientation of the cleavage plane is an actomyosin-dependent process [5] . Co-electroporation of cofilin S3A restored vertical cleavage-plane orientation in Rnd3 -silenced progenitors ( Fig. 2c ), thus indicating that Rnd3 maintains the vertical orientation of apical divisions by remodelling the actin cytoskeleton. 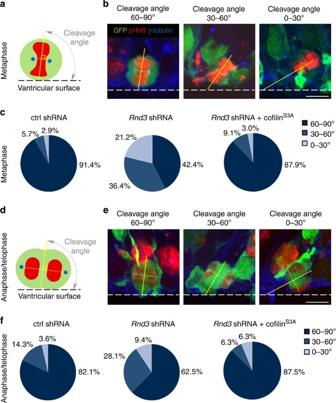Figure 2:Rnd3is required for vertical divisions of cortical progenitors. (a,d) The cleavage angles of electroporated (green) apical progenitors were measured during metaphase and ana-telophase as shown schematically inaandd, respectively. DNA is in red and centrosomes are in blue. (b,e) Cells in metaphase (b) and in anaphase/telophase (e) with vertical (60–90°), oblique (30–60°) or horizontal (0–30°) cleavage angles. Electroporated cells (GFP+) were labelled for phosphohistone H3 (pHH3) (mitotic cell, red) and γ-tubulin (centrosome, blue). The dashed line shows the ventricular surface. (c,f) Pie charts show the percentage of cells with colour-coded cleavage angles during metaphase (c) and ana- and telophase (f) 24 h after the electroporation (E14.5) of ctrl shRNA,Rnd3shRNA orRnd3shRNA+cofilinS3A. Metaphase: ctrl shRNAn=35 cells,Rnd3shRNAn=33 cells andRnd3shRNA+cofilinS3An=33 cells. Anaphase/telophase: ctrl shRNAn=20 cells,Rnd3shRNAn=22 cells andRnd3shRNA+cofilinS3An=32 cells. Cells were analysed from at least six embryos obtained from three litters. Scale bar, 5 μm. See also Supplementary Fig.S4. Figure 2: Rnd3 is required for vertical divisions of cortical progenitors. ( a , d ) The cleavage angles of electroporated (green) apical progenitors were measured during metaphase and ana-telophase as shown schematically in a and d , respectively. DNA is in red and centrosomes are in blue. ( b , e ) Cells in metaphase ( b ) and in anaphase/telophase ( e ) with vertical (60–90°), oblique (30–60°) or horizontal (0–30°) cleavage angles. Electroporated cells (GFP + ) were labelled for phosphohistone H3 (pHH3) (mitotic cell, red) and γ-tubulin (centrosome, blue). The dashed line shows the ventricular surface. ( c , f ) Pie charts show the percentage of cells with colour-coded cleavage angles during metaphase ( c ) and ana- and telophase ( f ) 24 h after the electroporation (E14.5) of ctrl shRNA, Rnd3 shRNA or Rnd3 shRNA+cofilin S3A . Metaphase: ctrl shRNA n =35 cells, Rnd3 shRNA n =33 cells and Rnd3 shRNA+cofilin S3A n =33 cells. Anaphase/telophase: ctrl shRNA n =20 cells, Rnd3 shRNA n =22 cells and Rnd3 shRNA+cofilin S3A n =32 cells. Cells were analysed from at least six embryos obtained from three litters. Scale bar, 5 μm. See also Supplementary Fig.S4. Full size image Rnd3 is required for the maintenance of adherens junctions Another mechanism that could account for the premature movement of Rnd3 -silenced cells out of the VZ is the loss of their junctions to neighbouring cells. Rnd3 expression in cortical progenitors is enriched at the ventricular surface (Fig. 6j), and Rnd3 has been implicated in the formation of tight junctions between epithelial tumour cells [35] . Moreover, Rnd3 regulates RhoA signalling in migrating neurons [26] , and RhoA is involved in the regulation of adherens junctions between progenitors in the cortical VZ and the spinal cord [17] , [18] , [19] . To investigate whether Rnd3 is required to maintain adherens junctions between radial glial cells, we examined the expression of components of adherens junctions in electroporated cortices. In Rnd3 -silenced cortices, expression of ZO1 was reduced and the ring-like distribution of β-catenin, N-cadherin and F-actin observed in control cortices was disrupted (compare Fig. 3a–d with Fig. 3e–h ; Supplementary Fig. S3 ). As with the other VZ progenitor defects described above, the expression and localization of junction markers was restored by co-electroporation of Rnd3 shRNA and cofilin S3A but not by co-electroporation of a mutant form of Rnd3 (Rnd3 T55V ) that cannot interact with p190RhoGAP and, therefore, does not inhibit RhoA signalling ( Fig. 3i–l and Supplementary Fig. S4 ). These results indicate that Rnd3 maintains the integrity of the junctions between radial glial cells through regulation of RhoA and the actin cytoskeleton. 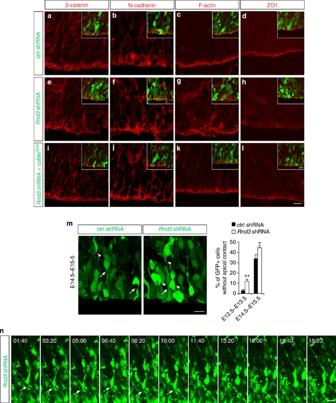Figure 3:Rnd3is required for the maintenance of adherens junctions. (a–l) Cortices immunostained for β-catenin (red ina,e,i), N-cadherin (red inb,f,j), F-actin (red inc,g,k) and ZO1 (red ind,h,l) 24 h after the co-electroporation at E14.5 of GFP (green) and ctrl shRNA (a–d),Rnd3shRNA (e–h) orRnd3shRNA+cofilinS3A(i–l). (m) Detachment of the apical process from the ventricular surface afterRnd3knockdown. White arrows and arrowheads indicate electroporated cells with and without an apical contact, respectively. The graph presents the quantification of the proportion of GFP+cells without an apical contact within 60 μm from the ventricle surface. E12.5–E13.5: ctrl shRNAn=239 cells andRnd3shRNAn=201 cells. E14.5–E15.5: ctrl andRnd3shRNAn=163 cells. Data represents the mean±s.e.m. from at least eight sections prepared from four embryos obtained from two or three litters. Student’st-test; *P<0.05 and **P<0.01. (n) Time-lapse series of a GFP+cell located into the upper part of the VZ analysed 24 h after electroporation (E14.5) ofRnd3shRNA, showing the retraction of the apical process after 11 h and 40 min of live imaging. White arrows indicate the apical process. Scale bar, 10 μm (land inset,m,n). See also Supplementary Figs S3, S4, S5 and Supplementary Movie 1. Figure 3: Rnd3 is required for the maintenance of adherens junctions. ( a – l ) Cortices immunostained for β-catenin (red in a , e , i ), N-cadherin (red in b , f , j ), F-actin (red in c , g , k ) and ZO1 (red in d , h , l ) 24 h after the co-electroporation at E14.5 of GFP (green) and ctrl shRNA ( a – d ), Rnd3 shRNA ( e – h ) or Rnd3 shRNA+cofilin S3A ( i – l ). ( m ) Detachment of the apical process from the ventricular surface after Rnd3 knockdown. White arrows and arrowheads indicate electroporated cells with and without an apical contact, respectively. The graph presents the quantification of the proportion of GFP + cells without an apical contact within 60 μm from the ventricle surface. E12.5–E13.5: ctrl shRNA n =239 cells and Rnd3 shRNA n =201 cells. E14.5–E15.5: ctrl and Rnd3 shRNA n =163 cells. Data represents the mean±s.e.m. from at least eight sections prepared from four embryos obtained from two or three litters. Student’s t -test; * P <0.05 and ** P <0.01. ( n ) Time-lapse series of a GFP + cell located into the upper part of the VZ analysed 24 h after electroporation (E14.5) of Rnd3 shRNA, showing the retraction of the apical process after 11 h and 40 min of live imaging. White arrows indicate the apical process. Scale bar, 10 μm ( l and inset, m , n ). See also Supplementary Figs S3, S4, S5 and Supplementary Movie 1. Full size image We then asked whether the disruption of adherens junctions between endfeets of radial glial progenitors was accompanied by a detachment of the apical process and premature delamination of the progenitors. We examined whether apical processes of GFP + -electroporated cells in the VZ contact the ventricular surface. We found that Rnd3 knockdown resulted in a higher proportion of VZ cells having an apical process detached from the ventricular surface ( Fig. 3m ), a defect also rescued by cofilin S3A co-electroporation ( Supplementary Fig. S5a ). VZ cells were also electroporated at E12.5 and examined at E13.5, a stage when delamination of radial glial cells is still infrequent. In control experiments, 3.0±0.8% of GFP + cells had an apical process that failed to reach the apical surface, and Rnd3 silencing increased this percentage to 12.1±2.0% ( Fig. 3m ). The premature detachment of the apical process was also observed by time-lapse imaging following Rnd3 knockdown but not in control sections ( Fig. 3n and Supplementary Movie 1 ). Therefore, Rnd3 activity is required to maintain adherens junctions between radial glial cells. The premature delamination of Rnd3 -silenced progenitors from the ventricular surface, revealed by the increased fraction of BrdU-labelled cells that move out of the VZ 6 h after the BrdU pulse ( Fig. 1g ), might thus be the result of the disruption of adherens junctions ( Fig. 3 ) and/or of the abnormal orientation of the cleavage planes of dividing VZ progenitors ( Fig. 2 ). Rnd3 regulates apical progenitor localization The premature detachment of radial glial cells from the ventricular surface could result in the displacement of apical progenitors (identified by Pax6 expression [36] ) and/or in their conversion to basal progenitors (identified by Tbr2 expression [37] ). Examination of Pax6 and Tbr2 expression in electroporated cells showed that the overall number of Pax6 + GFP + cells was not affected by Rnd3 knockdown ( Fig. 4b ). However, their distribution was altered, with more Pax6, GFP double-labelled cells present in the SVZ and IZ and fewer in the VZ than in control brains ( Fig. 4a ). This suggests that radial glial cells with impaired Rnd3 expression prematurely leave the VZ and enter the SVZ while transiently maintaining their radial glial molecular phenotype, and thus show similarities with outer radial glial [38] , [39] , [40] . Interestingly, this Rnd3 shRNA-induced displacement was prevented when cofilin S3A was co-electroporated ( Supplementary Fig. S5b,c ), indicating that it is actin dependent. Rnd3 knockdown also increased the fraction of GFP + cells expressing Tbr2 ( Fig. 4d ) and decreased the fraction expressing NeuN ( Fig. 4f ). Because the size of the Pax6 + population was not changed ( Fig. 4b ), the change in number of Tbr2 + cells might reflect an increased proliferation of basal progenitors rather than an effect of Rnd3 knockdown on the maturation of apical progenitors (see below). 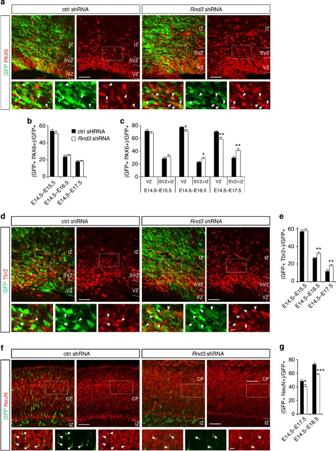Figure 4:Rnd3silencing results in translocation of apical progenitors to basal positions. (a,d,f) E17.5 cortices electroporated at E14.5 with ctrl shRNA orRnd3shRNA and immunostained for GFP (green) and the radial glial cell marker Pax6 (red ina), the basal progenitor marker Tbr2 (red ind) or the neuronal marker NeuN (red inf). White rectangles show the areas enlarged in the insets, and white arrowheads indicate double positive cells. (b,e,g) Percentage of electroporated cells that are PAX6+(b), or Tbr2+(e) or NeuN+(g). (c) The change in the proportion of GFP+PAX6+cells inside and outside the VZ shows thatRnd3silencing affects the location of apical progenitors. Data inb,c,e,gare presented as the mean±s.e.m. from at least six sections prepared from four embryos obtained from two or three litters. Student’st-test; *P<0.05, **P<0.01 and ***P<0.001. Scale bar, 10 μm (insetsa,d), 20 μm (insetf), 50 μm (a,d) and 100 μm (f). See also Supplementary Figs S4 and S5. Figure 4: Rnd3 silencing results in translocation of apical progenitors to basal positions. ( a , d , f ) E17.5 cortices electroporated at E14.5 with ctrl shRNA or Rnd3 shRNA and immunostained for GFP (green) and the radial glial cell marker Pax6 (red in a ), the basal progenitor marker Tbr2 (red in d ) or the neuronal marker NeuN (red in f ). White rectangles show the areas enlarged in the insets, and white arrowheads indicate double positive cells. ( b , e , g ) Percentage of electroporated cells that are PAX6 + ( b ), or Tbr2 + ( e ) or NeuN + ( g ). ( c ) The change in the proportion of GFP + PAX6 + cells inside and outside the VZ shows that Rnd3 silencing affects the location of apical progenitors. Data in b , c , e , g are presented as the mean±s.e.m. from at least six sections prepared from four embryos obtained from two or three litters. Student’s t -test; * P <0.05, ** P <0.01 and *** P <0.001. Scale bar, 10 μm (insets a , d ), 20 μm (inset f ), 50 μm ( a , d ) and 100 μm ( f ). See also Supplementary Figs S4 and S5. Full size image Rnd3 controls basal progenitor proliferation via cyclin D1 To determine whether Rnd3 regulates the proliferation of basal progenitors, we examined the expression of cell division markers. Rnd3 silencing significantly increased the number of cells expressing the mitotic marker phosphohistone H3 in the SVZ (where basal progenitors divide) but not in the VZ (where apical progenitors divide) ( Fig. 5a–c ). The fraction of cells expressing the proliferation marker Ki67 was also increased in the upper part of the VZ and the SVZ but not in the lower VZ ( Fig. 5d–f ). Moreover, time-lapse imaging showed that Rnd3 -silenced progenitors can undergo more than one round of division in the SVZ ( Supplementary Movie 2 ), which is uncommon in control brains [3] , [41] . Therefore, Rnd3 inhibits specifically the proliferation of basal progenitors. 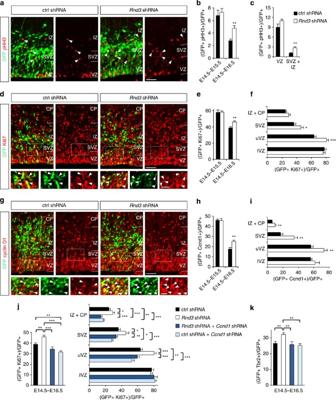Figure 5:Rnd3inhibits the proliferation of basal progenitors. (a,d,g) E16.5 cortices electroporated at E14.5 with ctrl shRNA orRnd3shRNA and immunostained for GFP (green) and phosphohistone H3 (pHH3) (red ina), GFP and Ki67 (red ind) or GFP and Ccnd1 (cyclin D1, red ing). White rectangles show the areas enlarged in the insets and white arrowheads indicate double positive cells. (b,e,h) Percentage of electroporated cells that are pHH3+(b), Ki67+(e) or Ccnd1+(h). (c,f,i) Quantification 2 days after electroporation of the percentage of electroporated cells that are pHH3+(c), Ki67+(f) or Ccnd1+(i) in the different zones of the cortex: lower VZ (lVZ), upper VZ (uVZ), SVZ, IZ and CP (cortical plate). Data inb,c,e,f,h,iare presented as the mean±s.e.m. from at least six sections prepared from four embryos obtained from two or three litters. Student’st-test; *P<0.05 and **P<0.01. (j,k) Co-electroporation ofCcnd1shRNA fully rescues the defects in proliferation, and Tbr2 expression was observed afterRnd3silencing. Data injandkare presented as the mean±s.e.m. one-way analysis of variance followed by a Fisher’s protected least significant differencepost-hoctest; *P<0.05, **P<0.01 and ***P<0.001. Scale bar, 20 μm (insetsd,g) and 50 μm (a,d,g). See also Supplementary Figs S4, S5 and Supplementary Movie 2. Figure 5: Rnd3 inhibits the proliferation of basal progenitors. ( a , d , g ) E16.5 cortices electroporated at E14.5 with ctrl shRNA or Rnd3 shRNA and immunostained for GFP (green) and phosphohistone H3 (pHH3) (red in a ), GFP and Ki67 (red in d ) or GFP and Ccnd1 (cyclin D1, red in g ). White rectangles show the areas enlarged in the insets and white arrowheads indicate double positive cells. ( b , e , h ) Percentage of electroporated cells that are pHH3 + ( b ), Ki67 + ( e ) or Ccnd1 + ( h ). ( c , f , i ) Quantification 2 days after electroporation of the percentage of electroporated cells that are pHH3 + ( c ), Ki67 + ( f ) or Ccnd1 + ( i ) in the different zones of the cortex: lower VZ (lVZ), upper VZ (uVZ), SVZ, IZ and CP (cortical plate). Data in b , c , e , f , h , i are presented as the mean±s.e.m. from at least six sections prepared from four embryos obtained from two or three litters. Student’s t -test; * P <0.05 and ** P <0.01. ( j , k ) Co-electroporation of Ccnd1 shRNA fully rescues the defects in proliferation, and Tbr2 expression was observed after Rnd3 silencing. Data in j and k are presented as the mean±s.e.m. one-way analysis of variance followed by a Fisher’s protected least significant difference post-hoc test; * P <0.05, ** P <0.01 and *** P <0.001. Scale bar, 20 μm (insets d , g ) and 50 μm ( a , d , g ). See also Supplementary Figs S4, S5 and Supplementary Movie 2. Full size image Rnd3 has previously been shown to inhibit cell-cycle progression in fibroblasts and glioblastoma cells [42] . Interestingly, this activity does not involve the regulation of RhoA/ROCK signalling as other functions of Rnd3, but the inhibition of cyclin D1 (Ccnd1) translation [43] , [44] , [45] . In agreement with these studies, we found that RhoA signalling and the actin cytoskeleton were not involved in the increase of basal progenitor proliferation observed after Rnd3 knockdown ( Supplementary Figs S4f–h and S5d–h ). We then examined Ccnd1 expression and found that Rnd3 silencing increased the number of Ccnd1 + cells in the upper VZ, SVZ and IZ of the cortex ( Fig. 5g–i ). Co-electroporation of a Ccnd1 shRNA construct [46] reduced the proliferation of Rnd3 -silenced progenitors to control levels, indicating that Rnd3 suppresses the proliferation of basal progenitors by inhibiting Ccnd1 expression ( Fig. 5j ). The increased number of Tbr2 + cells in Rnd3 -silenced cortices was also corrected by co-electroporation of Ccnd1 shRNA ( Fig. 5k ), indicating that this defect is due to an excessive proliferation of basal progenitors. The function and localization of Rnd3 are regulated by phosphorylation [47] , [48] . However, we showed previously that a non-phosphorylatable version of Rnd3, which is only expressed at the plasma membrane (Rnd3 All A ), could fully perform Rnd3 functions in migrating neurons [26] . Similarly, co-electroporation of Rnd3 All A with Rnd3 shRNA rescued the defects induced by Rnd3 knockdown in radial glial cells, including the non-vertical cleavage planes, the disruption of apical junctions and the increase in non-VZ Pax6+ cells ( Fig. 6a–d ). These results thus demonstrate that Rnd3 activities in radial glial cells do not require phosphorylation and indicate that Rnd3 is localized at the plasma membrane to mediate these functions ( Fig. 6j ). However, Rnd3 All A did not revert the excessive proliferation of SVZ progenitors or the increased number of Tbr2 + cells ( Fig. 6e–i ). This suggests that phosphorylation of Rnd3 is required for its function in basal progenitor proliferation. This result also confirms that Rnd3 uses distinct downstream mechanisms in radial glial cells (RhoA inhibition and depolymerization of actin filaments) and in basal progenitors (inhibition of cyclin D1 expression). 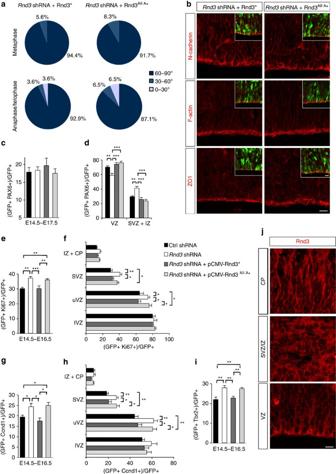Figure 6: Rnd3 activity in basal progenitor proliferation does not require its localization to the plasma membrane. (a) Rnd3* and Rnd3All A* restore cleavage-plane orientation inRnd3-deleted apical progenitors (the star indicates silent point mutations in the sequence recognized byRnd3shRNA). Pie charts show the percentage of cells with the colour-coded cleavage angle during metaphase and ana-telophase inRnd3shRNA+pCMV-Rnd3* (metaphasen=36 cells and ana/telophasen=28 cells) andRnd3shRNA+pCMV-Rnd3All A* cortices (metaphasen=36 cells and ana/telophasen=31 cells). (b) Immunostainings for N-cadherin, F-actin and ZO1 (in red) inRnd3shRNA+pCMV-Rnd3*, andRnd3shRNA+pCMV-Rnd3All A* electroporated cortices show no disruption of adherens junctions, similar to the pattern of expression observed in control sections. (c) Quantification of the percentage of electroporated cells that are PAX6+. (d) The quantification of the proportion of GFP+PAX6+cells inside and outside the VZ shows that Rnd3All A*restores the position of PAX6+progenitors afterRnd3knockdown. (e–i) However, Rnd3All A*does not rescue the increase of proliferation and basal progenitor population observed afterRnd3silencing, suggesting that Rnd3 is not localized at the plasma membrane to mediate these effects. (e–i) Quantification 2 days after the electroporation (E14.5) of the percentage of electroporated cells that are Ki67+(e), Ccnd1 (g) or Tbr2+ (i) in the entire electroporated cortex or in the different zones of the cortex (f,h). Data inc–iare presented as the mean±s.e.m; one-way analysis of variance followed by a Fisher’s protected least significant differencepost-hoctest; *P<0.05,**P<0.01 and***P<0.001. (j) Expression of Rnd3 in the different domains of the cerebral cortex at E15.5. In the VZ and CP, Rnd3 is essentially localized at the plasma membrane, whereas it is expressed throughout the cell in SVZ/IZ. Scale bar, 10 μm (band inset,j). Figure 6: Rnd3 activity in basal progenitor proliferation does not require its localization to the plasma membrane. ( a ) Rnd3* and Rnd3 All A * restore cleavage-plane orientation in Rnd3 -deleted apical progenitors (the star indicates silent point mutations in the sequence recognized by Rnd3 shRNA). Pie charts show the percentage of cells with the colour-coded cleavage angle during metaphase and ana-telophase in Rnd3 shRNA+pCMV-Rnd3* (metaphase n =36 cells and ana/telophase n =28 cells) and Rnd3 shRNA+pCMV-Rnd3 All A * cortices (metaphase n =36 cells and ana/telophase n =31 cells). ( b ) Immunostainings for N-cadherin, F-actin and ZO1 (in red) in Rnd3 shRNA+pCMV-Rnd3*, and Rnd3 shRNA+pCMV-Rnd3 All A * electroporated cortices show no disruption of adherens junctions, similar to the pattern of expression observed in control sections. ( c ) Quantification of the percentage of electroporated cells that are PAX6 + . ( d ) The quantification of the proportion of GFP + PAX6 + cells inside and outside the VZ shows that Rnd3 All A* restores the position of PAX6 + progenitors after Rnd3 knockdown. ( e – i ) However, Rnd3 All A* does not rescue the increase of proliferation and basal progenitor population observed after Rnd3 silencing, suggesting that Rnd3 is not localized at the plasma membrane to mediate these effects. ( e – i ) Quantification 2 days after the electroporation (E14.5) of the percentage of electroporated cells that are Ki67 + ( e ), Ccnd1 ( g ) or Tbr2+ ( i ) in the entire electroporated cortex or in the different zones of the cortex ( f , h ). Data in c – i are presented as the mean±s.e.m; one-way analysis of variance followed by a Fisher’s protected least significant difference post-hoc test; * P <0.05, ** P <0.01 and *** P <0.001. ( j ) Expression of Rnd3 in the different domains of the cerebral cortex at E15.5. In the VZ and CP, Rnd3 is essentially localized at the plasma membrane, whereas it is expressed throughout the cell in SVZ/IZ. Scale bar, 10 μm ( b and inset, j ). Full size image Ascl1 promotes vertical progenitor divisions via Rnd3 The expression of Rnd3 in the embryonic cerebral cortex is controlled transcriptionally by the proneural protein Ascl1. Moreover, Rnd3 mediates the function of Ascl1 in cortical neuron migration [26] . We thus asked whether Rnd3 also acts downstream of Ascl1 in cortical progenitors. We first determined whether Ascl1 inactivation results in similar progenitor defects as Rnd3 knockdown. Ascl1 silencing by electroporation of a specific shRNA or Ascl1 deletion in Emx1 Cre , Ascl1 flox/flox embryos resulted in an increase in the fraction of radial glial progenitors that divide with an oblique or horizontal cleavage plane ( Supplementary Fig. S6a,b ), a phenotype reminiscent of that of Rnd3 -silenced progenitors, although less pronounced ( Fig. 2c ). We then asked whether loss of Rnd3 contributes to this phenotype. Co-expressing Rnd3 with the Ascl1 shRNA rescued the division plane defect of Ascl1 -silenced progenitors ( Supplementary Fig. S6b ), demonstrating that Ascl1 maintains the vertical angle of radial glial cell divisions by inducing Rnd3 expression. In contrast with the increase in non-vertical divisions, Ascl1 knockdown or deletion did not produce other cellular defects observed in Rnd3- silenced progenitors, including delayed INM and disruption of adherens junctions ( Supplementary Fig. S7 ). Acute deletion of Ascl1 by electroporation of Cre in the cortical VZ of Ascl1 flox/flox embryos resulted in a reduction in the number of Ki67+ progenitors in the IZ ( Supplementary Fig. S6c,d ). This proliferation defect is similar to that observed in Ascl1 -deficient ventral telencephalon progenitors [49] , but it is opposite to that produced by Rnd3 knockdown ( Fig. 5d–f ). This is likely due to the regulation by Ascl1 of additional targets that regulate cell division in an opposite way to Rnd3 [49] . Extensive and dynamic remodelling of the cytoskeleton underlies many of the steps that dividing progenitors and newborn neurons go through during neurogenesis. We have previously shown that Rnd3, downstream of the proneural factor Ascl1, is a key factor in the regulation of neuronal migration in the embryonic cerebral cortex via its action on the actin cytoskeleton. In this study, we have asked (i) whether Rnd3 also regulates earlier steps of neurogenesis in the cerebral cortex, (ii) whether its activities in cortical progenitors involve actin remodelling and (iii) whether it acts downstream of Ascl1. Our results indicate that Rnd3 uses distinct downstream mechanisms in radial glial cells and in basal progenitors to mediate its pleiotropic functions ( Fig. 7 ). In radial glial cells, Rnd3 regulates the movement of the nuclei occurring during INM, exerts a control on the orientation of mitotic spindles and is required for the maintenance of adherens junctions. As for its function in migrating neurons [26] , Rnd3 regulates these different steps of neurogenesis by inhibiting actin filament polymerization. Indeed, the defects observed after Rnd3 knockdown were rescued when a constitutively active form of cofilin (cofilin S3A ) that disrupts actin filaments was co-electroporated. Reorganization of the actin cytoskeleton is known to drive cell rounding during mitosis, but the actin cortex has been shown to also guide mitotic spindle orientation through interactions with astral microtubules [5] , [50] . Our results suggest that the polymerization of actin filaments must be tightly regulated to maintain mitotic spindles aligned to the ventricular surface and that excessive polymerization perturbs the orientation of divisions. Interestingly, similar defects were observed in mice when LGN (the homologue of Partner of Inscuteable) was inactivated [1] . LGN is enriched in a ring located at the lateral cell cortex where it concentrates pulling forces on astral microtubules [51] . Rnd3 knockdown, by increasing cortical filamentous actin, might thus prevent the anchoring or the correct distribution of LGN complex and, consequently, proper spindle positioning. In migrating neurons, Rnd3 promotes actin cytoskeleton remodelling by inhibiting RhoA signalling at the plasma membrane through stimulation of the Rho GTPase-activating protein p190RhoGAP [26] . We used an in vivo rescue assay with mutated forms of Rnd3 that cannot interact with p190RhoGAP (Rnd3 T55V ) or that is only expressed at the plasma membrane (Rnd3 All A ), to show that Rnd3 uses a similar mechanism in apical progenitors to regulate actin-dependent processes ( Fig. 6 and Supplementary Fig. S4a–e ). 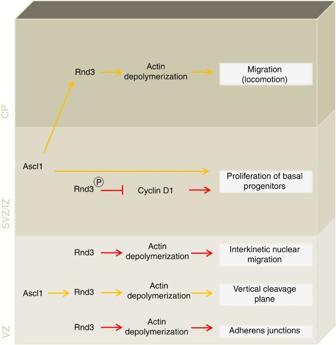Figure 7: Roles of Rnd3 in cortical neurogenesis. In radial glial cells, Rnd3 regulates INM, exerts a control on the orientation of the mitotic spindles and maintains the adherens junctions by inhibiting actin filament polymerization. In basal progenitors, Rnd3 controls proliferation through cyclin D1. Rnd3 also regulates migration of postmitotic neurons via its action on the actin cytoskeleton. See also Supplementary Figs. S6 and S7. Figure 7: Roles of Rnd3 in cortical neurogenesis. In radial glial cells, Rnd3 regulates INM, exerts a control on the orientation of the mitotic spindles and maintains the adherens junctions by inhibiting actin filament polymerization. In basal progenitors, Rnd3 controls proliferation through cyclin D1. Rnd3 also regulates migration of postmitotic neurons via its action on the actin cytoskeleton. See also Supplementary Figs. S6 and S7. Full size image Adherens junctions interact with circumferential actin filaments bundles, via the α-catenin component of cadherin–catenin complexes and other actin-binding proteins, and these interactions are essential for the development, remodelling and function of the junctions [7] , [52] , [53] . Small GTPases are recruited and activated at adherens junctions and have a pivotal role in the dynamic remodelling of the junctions [18] , [53] , [54] . In particular, RhoA and its downstream effector mDia1 control the localization and stabilization of cadherin–catenin complexes at the junctions by mediating their association to the cortical actin cytoskeleton [6] , [17] , [19] . Interestingly, excessive RhoA activity in colon carcinoma and non-tumorigenic epithelial cells results in contraction of the actomyosin cytoskeleton and disruption of adherens junctions, an effect mediated by another downstream RhoA effector, ROCK [6] . If RhoA has similar activities in the cortical neuroepithelium, then Rnd3 may maintain the integrity of adherens junctions by moderating the level of RhoA-ROCK signalling, thus preventing excessive contraction of the actomyosin cytoskeleton. Rnd3 knockdown also increased the number of Tbr2 + cells. This effect did not occur at the expense of Pax6 + progenitor cells, suggesting that it is the result of excessive proliferation rather than of a change of progenitor fate. Accordingly, Rnd3 silencing resulted in an increase in the number of cells expressing cyclin D1 and the mitotic marker Ki67 + , particularly in the upper VZ and SVZ where basal progenitors are located. Rnd3 inhibits cell-cycle progression in fibroblasts and glioblastoma cells independently of the inhibition of RhoA/ROCK signalling, by interfering with the release of the eukaryotic initiation factor eIF4E from the translation repressor 4E-BP1, resulting in the suppression of cyclin D1 translation [43] , [44] , [45] . Similarly, we found that the silencing of cyclin D1 together with Rnd3 eliminated the supernumerary Ki67 + and Tbr2 + cells. Therefore, our results demonstrate that Rnd3 limits the proliferation of Tbr2 + basal progenitors independently of the RhoA-actin pathway but through regulation of cyclin D1 expression, in agreement with earlier work demonstrating the importance of cyclin D1 regulation in controlling the rate of generation and expansion of basal progenitors [46] . Rnd3 expression in cortical progenitors and postmitotic neurons is controlled transcriptionally by the proneural protein Ascl1, and Rnd3 acts downstream of Ascl1 in the regulation of cortical neuron migration [26] . Our finding that Ascl1 inactivation in cortical progenitors has more limited effects than Rnd3 knockdown was therefore unexpected. Elimination of Ascl1 altered the orientation of the mitotic spindles in dividing radial glial, a defect corrected by expression of Rnd3 . Thus, Ascl1 promotes vertical divisions in the cortical VZ mainly by modulating the actin cytoskeleton via Rnd3 regulation. However, we did not observe defects in INM or in adherens junction integrity when Ascl1 was inactivated as when Rnd3 is silenced. One hypothesis is that loss of Ascl1 does not completely abolish Rnd3 expression in the VZ [26] , and the different Rnd3 -dependent processes could be differently sensitive to reduced Rnd3 levels. A moderate decrease of Rnd3 expression after Ascl1 inactivation may not have an impact INM and junctions but may affect the orientation of the cleavage plane. Another possible explanation for the discrepancy between Rnd3 knockdown and Ascl1 knockdown/knockout results is that Ascl1 inactivation modifies the expression of other targets of Ascl1 that act in an opposite direction from Rnd3 and thus compensate the effect of Rnd3 silencing on INM and adherens junctions. These targets might not regulate cleavage-plane orientation. Moreover, Ascl1 inactivation resulted in a decrease in proliferation in the IZ and CP, that is, an opposite phenotype from that of Rnd3 knockdown. Ascl1 has been shown to induce the expression of cell cycle-promoting genes, such as E2f1 and Cdk1/2, in the ventral telencephalon and in cultivated neural stem cells [49] . If these genes are also regulated by Ascl1 in the cortex, the net effect of their downregulation and that of Rnd3 when Ascl1 is inactivated might be a slowdown of divisions. The identification and analysis of additional targets of Ascl1 in cortical progenitors will allow us to test this hypothesis. Animals Mice were housed, bred and treated according to the guidelines approved by the Home Office under the Animal (Scientific procedures) Act 1986. The following mouse lines were used and genotyped as described previously: Ascl1 flox [26] and Emx1 Cre [55] . In utero electroporation and tissue processing In utero electroporation of the cerebral cortex was performed as described previously [56] . A concentration of 1 μg μl −1 was used for each construct. The different expression plasmids and shRNA constructs used have been described previously [26] . CyclinD1 shRNA was a kind gift from Dr Federico Calegari [46] . At the desired time point after electroporation, pregnant mice were killed by neck dislocation and embryos were processed for tissue analyses. Embryonic brains were fixed in 4% PFA overnight and then placed in 20% sucrose/PBS overnight. Embryonic brains were then embedded in OCT compound and frozen before sectioning using a cryostat. Immunostaining After washing in PBS, sections were treated with PBS–0.01% Triton X-100–10% serum for 30 min. They were then incubated overnight at 4 °C with the following primary antibodies diluted in the blocking buffer: rat anti-BrdU (1/1000; AbD Serotec), rabbit anti-cyclinD1 (1/25; Thermo Fisher Scientific), chicken anti-GFP (1/700; Millipore), mouse anti-Ki67 (1/50; BD Pharmingen), mouse anti-NeuN (1/1000; Millipore), rabbit anti-PAX6 (1/200; Covance), rabbit anti-pHH3 (1/200; Upstate), mouse anti-Rnd3 (1/500; Abcam), rabbit anti-Tbr2 (1/500; Abcam) and mouse anti γ-tubulin (1/100; Abcam). Sections were then incubated with appropriate fluorescent secondary antibodies. Pretreatment with 2 N HCl for 30 min at 37 °C before pre-incubation with primary antibody was performed to detect BrdU. To detect NeuN, a step of antigen retrieval with citrate was performed before the blocking (sodium citrate pH=6 for 15 min at 90 °C). The junctional markers were immunostained as described previously [57] with minor modifications. After 5 min in PBS–1% Triton X-100, sections were treated with a blocking buffer containing PBS–1% Triton X-100 and bovine serum albumin (3%) for 1 h. Primary antibodies were incubated overnight at room temperature in the blocking buffer without detergent: rabbit anti β-catenin (1/800; Sigma), mouse anti N-cadherin (1/100; BD Transduction Laboratories) and rabbit anti ZO1 (1/200; Zymed). Appropriate fluorescent secondary antibodies diluted in PBS were incubated for 1 h. F-actin filaments were visualized using rhodamine-labelled phalloidin (Sigma). Sections were permeabilized 10 min with 0.1% Triton X-100-PBS, incubated with rhodamine-labelled phalloidin diluted in PBS (0.2 μg ml −1 ) for 40 min and washed several times in PBS. All images were acquired with a laser scanning confocal microscope (Radiance 2100; Bio-Rad). Cell counts were performed using MetaMorph software (Molecular Devices). BrdU labelling Interkinetic nuclear migration . Cerebral cortices were electroporated in utero at E14.5 and subjected to 30 min, 3 h or 6 h BrdU (50 mg kg −1 ) pulse labelling 24 h after the electroporation. After the pulse, co-immunostaining for GFP and BrdU was performed. The cortex was then divided into bins of 20 μm in height, and the proportion of GFP+/BrdU+ cells was determined in each bin with bin 1 at the ventricle surface. Labelling index Cerebral cortices were electroporated ex vivo at E14.5 as previously described [26] . After two DIV, BrdU (final concentration of 20 μg ml −1 ) was added every 10 h. Sections were fixed 1, 3.5, 5.5, 8 and 11.5 h after the first addition of BrdU. Measure of G1 duration To measure G1-phase duration in the electroporated population in vivo , BrdU pulse injection (30 min, 50 mg kg −1 ) was performed 8, 10, 12, 14 and 16 h after in utero electroporation at E14.5 as previously described [58] . The percentage of electroporated (GFP + ) cells that had incorporated BrdU was then determined at the different time points. Live imaging One day after ex vivo electroporation, GFP was imaged in live brain slices using 900 nm multiphoton excitation (Spectra-Physics; DeepSee) with a Leica SP5 confocal scanner on a DM6000 CFS upright microscope. A × 10, 0.4 NA (dry) lens was used, and reflected excitation was collected with a non-descanned PMT through a 525/50 filter (Chroma). Statistical analysis A statistical analysis was performed using either unpaired two-tailed Student’s t -test between control and experimental condition or one-way analysis of variance followed by a Fisher’s protected least significant difference post-hoc test for multiple comparisons (StatView software, version 5). Details for each experiment are described in figure legends. How to cite this article: Pacary, E. et al . Rnd3 coordinates early steps of cortical neurogenesis through actin-dependent and -independent mechanisms. Nat. Commun. 4:1635 doi: 10.1038/ncomms2614 (2013).